Rift migration explains continental margin asymmetry and crustal hyper-extension When continents break apart, continental crust and lithosphere are thinned until break-up is achieved and an oceanic basin is formed. The most remarkable and least understood structures associated with this process are up to 200 km wide areas of hyper-extended continental crust, which are partitioned between conjugate margins with pronounced asymmetry. Here we show, using high-resolution thermo-mechanical modelling, that hyper-extended crust and margin asymmetry are produced by steady state rift migration. We demonstrate that rift migration is accomplished by sequential, oceanward-younging, upper crustal faults, and is balanced through lower crustal flow. Constraining our model with a new South Atlantic plate reconstruction, we demonstrate that larger extension velocities may account for southward increasing width and asymmetry of these conjugate magma-poor margins. Our model challenges conventional ideas of rifted margin evolution, as it implies that during rift migration large amounts of material are transferred from one side of the rift zone to the other. The extensively surveyed Iberia/Newfoundland and Angola/Brazil conjugates provide detailed information on magma-poor rifted margin formation. They exhibit hyper-extended (with a thickness <10 km) crustal slivers that vary in widths between 70 km offshore Iberia [1] , [2] and 200 km off Angola [3] . The respective conjugate margin width, however, is restricted to a few tens of kilometres [4] , [5] , resulting in large-scale crustal asymmetry. Observations off Iberia indicate that brittle deformation is accommodated by sequentially active normal faults [2] , with very thin syn-rift deposits supporting short-lived individual fault activity, that is, in the order of a few million years [2] , [6] . Similarly, the wide South Atlantic margins feature undeformed, pre-break-up sediments [5] , [7] below Aptian salt deposits [8] , which requires that extensive local rift activity, achieving crustal thinning of a factor larger than 3, was surprisingly restricted to a few million years and did not result in break-up at this location. Despite great academic and economic interest in hyper-extended margins and instructive field-based studies [1] , [2] , [3] , [4] , [5] , [6] , [9] , [10] , [11] , no suitable thermo-mechanically corroborated model has been presented so far. A previous numerical model [12] is problematic for several reasons: it suggests that the crust is thinned by permanent pure shear both at the proximal and distal margin; a scenario that is contradicted by observations of undisturbed, pre-break-up sediments along the African margin. A felsic flow law for the entire crust is used that is not supported by the seismically inferred mafic (that is, strong) composition of the lower crust [3] . Finally, the previous study [12] produced symmetric margins and could not explain the dominant asymmetry of the South Atlantic and Iberia/Newfoundland conjugate margins. In this study, we propose rift migration as a key process during hyper-extended margin formation. Our numerical models indicate that steady-state rift migration is maintained by sequential faulting in the brittle crust and controlled by lower crustal flow. Thus, the extent of rift migration depends on lower crustal viscosity near the moving rift, which in turn is a function of extension velocity, lower crustal composition, intensity of strain softening and initial thermal structure. By demonstrating how lower crustal viscosity and the rate of extension affect the final margin width, we explain the formation of hyper-extended crust and the degree of asymmetry in the Central South Atlantic and Iberia/Newfoundland within a single model framework. Initiation and dynamic maintenance of rift migration We use thermo-mechanical finite-element models to investigate lithospheric thinning. The applied rheologies, initial temperature fields and extension velocities are discussed in the Methods section, while a setup sketch and all model parameters are provided in Supplementary Fig. 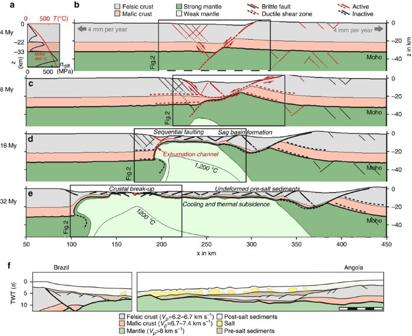Figure 1: The process of steady-state rift migration. (a–e) Fault kinematics of the model. Active faults are shown in red and inactive faults in black. Brittle faults are indicated with solid lines, ductile shear zones with dashed lines. The wide margin is formed through rift migration and sequentially active faulting towards the future ocean. Hence, thick undisturbed pre-salt sediments pre-dating break-up are predicted by our model to be deposited in the landward part of the margin (d,e). The final crustal structure of the model reproduces the strong asymmetry (f) of the conjugate Campos Basin–Angola margins (modified after ref.5). Note that the geosection is drawn without vertical exaggeration at the same scale as the model (scale bar in the lower right corner is 50 km long). Vertical scale is in seconds two-way travel time (TWT). 1 and Supplementary Table 1 , respectively. Modelled rift evolution is shown in Figs 1 and 2 . Rifting starts with a fault network that distributes deformation across the whole width of the model before friction softening causes coalescence [13] into a dominant single fault with few antithetic faults [14] , which is typical for narrow rifts such as the East African Rift System [15] . The time necessary for the deformation to localize into this dominant fault is a function of lower crustal rheology, with weaker rheologies showing a more prolonged phase of initial distributed faulting. At the downward tip of this normal fault, brittle and ductile deformation in crust and mantle are strongly linked. Hence, slip along the dominant initial fault results in severe lithospheric thinning and hot asthenospheric upwelling. Simultaneously, sub-horizontal ductile shear zones develop in the lower portions of both the felsic and mafic crust ( Figs 1c and 2b ) as described for the South Atlantic conjugates [10] , the Iberian margin [16] and in previous numerical rift simulations [17] . Figure 1: The process of steady-state rift migration. ( a – e ) Fault kinematics of the model. Active faults are shown in red and inactive faults in black. Brittle faults are indicated with solid lines, ductile shear zones with dashed lines. The wide margin is formed through rift migration and sequentially active faulting towards the future ocean. Hence, thick undisturbed pre-salt sediments pre-dating break-up are predicted by our model to be deposited in the landward part of the margin ( d , e ). The final crustal structure of the model reproduces the strong asymmetry ( f ) of the conjugate Campos Basin–Angola margins (modified after ref. 5 ). Note that the geosection is drawn without vertical exaggeration at the same scale as the model (scale bar in the lower right corner is 50 km long). Vertical scale is in seconds two-way travel time (TWT). 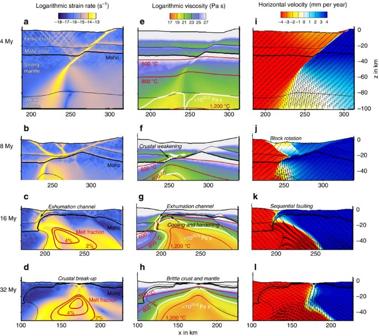Figure 2: Key variables of the numerical model. Shown are (a–d) strain rate, (e–h) viscosity and (i–l) horizontal velocity. A dominant fault at 4 My induces asymmetric hot mantle upwelling and subsequent asymmetric lower crustal weakening (a). A low-viscosity crustal pocket forms at the tip of sequential upper crustal faults, together forming the ‘exhumation channel’ that is visible in terms of high strain rate (c) and low viscosity (g). The existence of the low-viscosity pocket facilitates lower crustal flow towards the down-dip fault end rendering fault-induced Moho uplift less efficient. Rift migration is caused by a lateral strength gradient between the low-viscosity pocket and the cooling mantle at the fault’s footwall. Rift migration stops when the lower crust becomes more viscous, followed by crustal embrittlement (h), and soon after crustal break-up takes place. Full extension velocity is 8 mm per year. Note that grey regions in (e–h) where viscosity is maximal, deform via brittle behaviour. The depicted x-interval varies between time steps, as shown inFig. 1. For detailed model evolution, see animated strain rate and viscosity plots inSupplementary Fig. 3. Full size image Figure 2: Key variables of the numerical model. Shown are ( a – d ) strain rate, ( e – h ) viscosity and ( i – l ) horizontal velocity. A dominant fault at 4 My induces asymmetric hot mantle upwelling and subsequent asymmetric lower crustal weakening ( a ). A low-viscosity crustal pocket forms at the tip of sequential upper crustal faults, together forming the ‘exhumation channel’ that is visible in terms of high strain rate ( c ) and low viscosity ( g ). The existence of the low-viscosity pocket facilitates lower crustal flow towards the down-dip fault end rendering fault-induced Moho uplift less efficient. Rift migration is caused by a lateral strength gradient between the low-viscosity pocket and the cooling mantle at the fault’s footwall. Rift migration stops when the lower crust becomes more viscous, followed by crustal embrittlement ( h ), and soon after crustal break-up takes place. Full extension velocity is 8 mm per year. Note that grey regions in ( e – h ) where viscosity is maximal, deform via brittle behaviour. The depicted x-interval varies between time steps, as shown in Fig. 1 . For detailed model evolution, see animated strain rate and viscosity plots in Supplementary Fig. 3 . Full size image Upwelling of hot mantle material is more pronounced near the down-dip end of the initial dominant fault, so that the 600 °C isotherm penetrates into the lower crust. Elevated temperature and viscous strain softening generate a pocket of weak lower crust at the fault tip (see white isoviscosity line of 10 20.5 Pa s in Fig. 2f,g ). In analogy to the subduction channel at convergent plate boundaries, we refer to this weak locus of deformation as ‘exhumation channel’. At the footwall side of the exhumation channel where the upwelling mantle is shallowest, cooling and strengthening of mantle material takes place [18] , [19] ( Fig. 2g ). These two processes—softening at the tip of the active fault and strengthening at its footwall—generate a lateral strength gradient that forces migration of the rift in a steady-state manner. During migration, new rift-bounding faults are generated that become sequentially active. Ductile lower crust flows within the exhumation channel towards the down-dip end of any of these faults ( Fig. 3h,i ). This flow balances the faults’ tendency for crustal thinning and break-up, and it promotes the formation of a single, wide margin on one rift side with crust thinned to a thickness of <10 km. Opposite to previous models of margin formation [20] , [21] , we find that large-scale asymmetry does not form by slip on large detachment faults cross-cutting the crust or entire lithosphere, but by an array of oceanward dipping faults that act sequentially in time [2] . 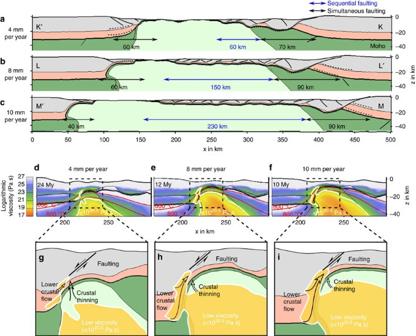Figure 3: Influence of rift velocity. (a–c) Conjugate margin structure for 4, 8 and 10 mm per year full rift velocities. The width of simultaneously faulted areas is indicated by black arrows, whereas sequentially faulted domains are depicted by blue arrows. The width of the wide margin increases with rift velocity. The reason for this behaviour is shown ind–f: Higher velocities lead to advection of the isotherms to shallower depths. This heats the lower crust more efficiently, forming a weaker and larger exhumation channel. (g–i) Facilitated lower crustal flow counteracts fault-controlled crustal thinning and prolongs the phase of rift migration leading to a wider margin. For animated model evolution, seeSupplementary Fig. 3 Figure 3: Influence of rift velocity. ( a – c ) Conjugate margin structure for 4, 8 and 10 mm per year full rift velocities. The width of simultaneously faulted areas is indicated by black arrows, whereas sequentially faulted domains are depicted by blue arrows. The width of the wide margin increases with rift velocity. The reason for this behaviour is shown in d – f : Higher velocities lead to advection of the isotherms to shallower depths. This heats the lower crust more efficiently, forming a weaker and larger exhumation channel. ( g – i ) Facilitated lower crustal flow counteracts fault-controlled crustal thinning and prolongs the phase of rift migration leading to a wider margin. For animated model evolution, see Supplementary Fig. 3 Full size image During migration of the rift centre, previously active faults are abandoned, whereas new faults form on top of the exhumation channel cutting into undisturbed crust of the left-hand rift side. This accretes crustal material across the migrating plate boundary zone (white region in Fig. 2i–l ) to the opposite rift side. Therefore, in contradiction to the common assumption that the stretched continental crust of a passive margin consists of deformed material of the same plate, our model suggests that large parts of a hyper-extended margin originate from the formerly opposite side of the rift zone. Despite extreme final margin widths of more than 200 km ( Fig. 1e ), the actively deforming plate boundary zone appears to be very narrow (~\n30 km; Fig. 2c ). Crustal thinning in the rift is accomplished by short-lived (a few million years) sequential faults with high-slip velocities (for example, 12 mm per year slip on the fault plane for 8 mm per year full extension velocity). This implies limited available time for syn-rift sediment to accumulate and agrees well with observations off West Iberia [2] , [6] . At very wide margins that experience a long period of rift migration (such as the Angolan Kwanza Basin), the proximal part of the margin exhibits undisturbed sedimentary successions that are dominated by thermal subsidence [5] , [7] , although their age is actually pre-break-up [22] . Moreover, lateral motion of the rift centre causes oceanward migrating peak heat flow, with strong implications for hydrocarbon maturation patterns. With continued rift migration, the steady-state heat supply to the exhumation channel decreases. The crust becomes cooler, and the ductile portions of the crust strengthen to a degree that the low-viscosity pocket vanishes. The crust becomes progressively brittle and faults penetrate into the mantle (as suggested for West Iberia [1] , [23] ). Soon after, these faults bring the crust to break-up until mantle is exhumed with very little magmatic activity ( Fig. 2d ). Influence of rift velocity The longevity of the exhumation channel, and hence the final width of the conjugate margins, is determined by the ability of the lower crust to flow into the area where active faults terminate at depth. This replenishing of lower crust depends on the lower crustal viscosity and hence on temperature distribution, crustal rheology and the operating weakening mechanisms. High rift velocities lead to more efficient heat advection and thus elevate the temperature of the exhumation channel ( Fig. 3 ). The extent of the low-viscosity pocket is increased ( Fig. 3d–f ) and rift migration is maintained over a longer distance. Hence, faster extension results in wider margins with more pronounced asymmetry. The conjugate South Atlantic margins of the central segment are an excellent test case for this model prediction as intraplate deforming zones in Africa allow to robustly reconstruct the pre-break-up kinematic history of the South Atlantic Rift [24] , [25] . The stage poles describing initial extension and early seafloor spreading history are located close to the northern tip of the South Atlantic Rift. Consequently, relative plate velocities between Africa and South America increase away from the stage pole, resulting in extensional velocities increasing southward along strike of the South Atlantic Rift system ( Fig. 4a ). This inference is also robustly featured in other reconstructions [8] , [26] , [27] , [28] . Independent evidence for opening velocities comes from seismic section restoration at the Campos and Camamu basins (M. Araujo, personal communication) yielding extension rates that correspond well with the plate kinematic model. 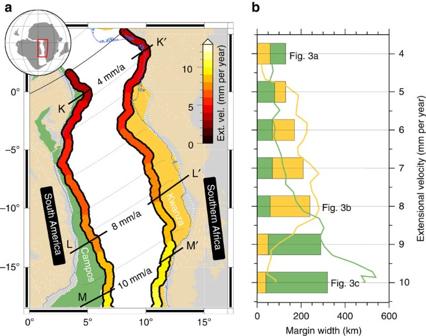Figure 4: Central South Atlantic extension velocities and margin width. (a) The Central South Atlantic segment shown in a post-break-up configuration. Extended continental crust coloured by plate (Africa: orange and South America: green). Landward limit of oceanic crust or continent–ocean boundary is defined by extensive mapping using industry-quality seismic reflection data in conjunction with high-resolution potential field data24. It is coloured by extension velocities (Ext. vel.) that are computed using the 127–140 Ma stage pole for South America relative to a fixed African plate. Margin widths are measured in km along flowlines (thin dashed lines). (b) Margin width versus extension velocity for numerical model (bars) and plate kinematic reconstruction (lines) for African (orange) and South American margins (green). In agreement with the numerical model, the width of the wider margin increases almost linearly with rift velocity. All velocities refer to full extension rates. Margin width of the numerical model (bars) represents the sum of simultaneously and sequentially faulted areas (Fig. 3). Both the green and the orange bars start from zero; that is, the bar plot is not cumulative. Figure 4: Central South Atlantic extension velocities and margin width. ( a ) The Central South Atlantic segment shown in a post-break-up configuration. Extended continental crust coloured by plate (Africa: orange and South America: green). Landward limit of oceanic crust or continent–ocean boundary is defined by extensive mapping using industry-quality seismic reflection data in conjunction with high-resolution potential field data [24] . It is coloured by extension velocities (Ext. vel.) that are computed using the 127–140 Ma stage pole for South America relative to a fixed African plate. Margin widths are measured in km along flowlines (thin dashed lines). ( b ) Margin width versus extension velocity for numerical model (bars) and plate kinematic reconstruction (lines) for African (orange) and South American margins (green). In agreement with the numerical model, the width of the wider margin increases almost linearly with rift velocity. All velocities refer to full extension rates. Margin width of the numerical model (bars) represents the sum of simultaneously and sequentially faulted areas ( Fig. 3 ). Both the green and the orange bars start from zero; that is, the bar plot is not cumulative. Full size image We find that the maximum width of the conjugate margin cross-sections increases southward almost linearly ( Fig. 4b ). Similarly, numerical models with varied extensional velocities exhibit a southward increase in hyper-extended margin width. In particular, our modelling indicates a linear relationship between extension velocity and margin width ( Figs 3a–c and 4b ). Although the polarity of the South Atlantic hyper-extended margins alternates, the width of the wider margin is very well reproduced by the numerical results. Note that the reason for the polarity switch cannot be addressed within our two-dimensional (2D) model framework. Similarly, the evolution of the Santos basin, south of Campos, that is characterized by a complicated three-dimensional tectonic and magmatic evolution [29] lies outside of our 2D modelling scope. Influence of initial thermal profile Lower crustal temperatures and rheology jointly affect the lower crustal viscosity and the depth of the crustal brittle-ductile transition. A cold, strong crust with a thick brittle layer effectively couples brittle deformation of crust and mantle through thin ductile shear zones producing a narrow rift [30] ( Fig. 5g ). Fault and shear zone weakening results in strong competition between faults, producing a single master fault in a simple shear system that leads to strong rift asymmetry [14] , [31] . Hot, weak lower crust, on the other hand, decouples brittle deformation between crust and mantle generating a wide rift [30] that eventually generates symmetric, wide margins [32] (see Supplementary Discussion , Supplementary Fig. 2 and Supplementary Table 2 ). 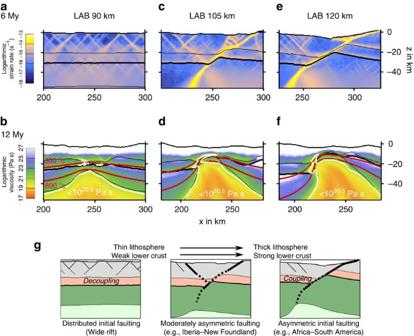Figure 5: Influence of initial thermal profile. (a,b) Thin (90 km) and hence hot lithosphere favours crust–mantle decoupling, pure shear deformation and distributed faulting without rift migration. (c,d) For intermediate depth of the lithosphere–asthenosphere boundary (LAB) initially pure shear straining with moderately asymmetric faulting generates a small low-viscosity pocket and a short rift migration phase. (e,f) For comparison, model results are shown with an LAB thickness of 120 km (as inFig. 1) that involve strong crust–mantle coupling and generate a large low-viscosity pocket. Full extension velocity is 8 mm per year. We use the 1,300 °C isotherm to define the thermal LAB. Detailed model evolution is animated inSupplementary Fig. 3. (g) Cartoon illustrating how lithosphere thickness and crust–mantle decoupling affect initial fault pattern. Figure 5: Influence of initial thermal profile. ( a , b ) Thin (90 km) and hence hot lithosphere favours crust–mantle decoupling, pure shear deformation and distributed faulting without rift migration. ( c , d ) For intermediate depth of the lithosphere–asthenosphere boundary (LAB) initially pure shear straining with moderately asymmetric faulting generates a small low-viscosity pocket and a short rift migration phase. ( e , f ) For comparison, model results are shown with an LAB thickness of 120 km (as in Fig. 1 ) that involve strong crust–mantle coupling and generate a large low-viscosity pocket. Full extension velocity is 8 mm per year. We use the 1,300 °C isotherm to define the thermal LAB. Detailed model evolution is animated in Supplementary Fig. 3 . ( g ) Cartoon illustrating how lithosphere thickness and crust–mantle decoupling affect initial fault pattern. Full size image In between these two end members, intermediate crust–mantle coupling generates a moderately asymmetric fault pattern [14] , [17] . We analyse how the initial lower crustal strength influences rift migration and ultimately margin geometry by varying the initial depth of the thermal lithosphere–asthenosphere boundary (LAB; the 1,300 °C isotherm) between 90 km ( Figs 5a,b and 6a ), 105 km ( Figs 5c,d and 6b ) and 120 km ( Figs 1e and 5e,f ). We find that initial fault symmetry impedes rift migration while a singular normal fault leads to asymmetric mantle upwelling, which heats its hanging wall producing a low-viscosity exhumation channel enhancing rift migration. Hence, the initial fault pattern controls the extent of simultaneously and sequentially faulted areas ( cf . blue and black arrows in Figs 3a–c and 6a,b ). We note that other combinations of rheology and lithospheric thickness, as long as they result in similar lower crustal viscosity and brittle layer thickness, lead to a qualitatively identical rift evolution. 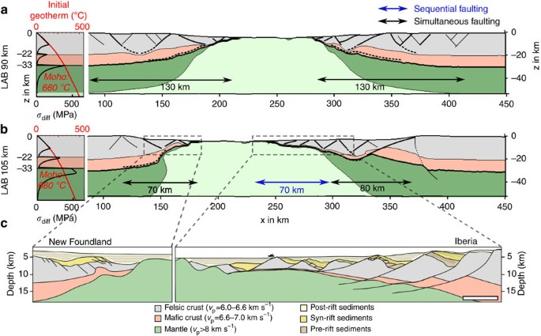Figure 6: Final margin widths for different initial thermal profiles. (a) Scenario with 90 km thick thermal lithosphere. Owing to crust–mantle decoupling (Fig. 5) symmetric rifting takes place without rift migration. (b) The setup with 105 km thick lithosphere generates a distinct rift migration phase. The width of simultaneously faulted areas is indicated by black arrows, whereas sequentially faulted domains are depicted by blue arrows. The model inbis comparable tocthe Iberia–Newfoundland conjugates (modified after ref.2). This geosection is drawn without vertical exaggeration and the scale bar in the lower right corner is 10 km long. Figure 6: Final margin widths for different initial thermal profiles. ( a ) Scenario with 90 km thick thermal lithosphere. Owing to crust–mantle decoupling ( Fig. 5 ) symmetric rifting takes place without rift migration. ( b ) The setup with 105 km thick lithosphere generates a distinct rift migration phase. The width of simultaneously faulted areas is indicated by black arrows, whereas sequentially faulted domains are depicted by blue arrows. The model in b is comparable to c the Iberia–Newfoundland conjugates (modified after ref. 2 ). This geosection is drawn without vertical exaggeration and the scale bar in the lower right corner is 10 km long. Full size image The Iberia–Newfoundland rift is best described with intermediate lithosphere thickness of 105 km ( Fig. 6b,c ), where an initially decoupled, moderately asymmetric fault phase is followed by crust–mantle coupling, sequential faulting and low-degree rift migration [33] (see also Supplementary Fig. 3 ). Our thermal setup is supported by lithospheric thickness estimates that are generally lower for Iberia–Newfoundland than for Africa–South America [34] . We compare our results with previous numerical studies on rifted margin formation. During the initial extension phase, our models agree with an earlier study [14] only that viscous strain softening in our model is considerably smaller and their models stop before hyper-extension takes place. The model with slow extension (4 mm per year; Fig. 3a ) evolves very similar to previous work [17] , [35] , generating moderately asymmetric margins. However, in our models, it is not a concave-downward detachment fault that generates the wide margin, but short-lived, sequentially active normal faults that accomplish lateral rift migration as imaged on seismic data [2] . Note that our explanation for crustal hyper-extension strongly differs from that of a previous study [12] , where the crust is thinned by permanent pure shear both at the proximal and distal margin and no pronounced asymmetry is generated (see comparable scenario in Supplementary Fig. 2c,f and Supplementary Fig. 4 ). We conclude that steady-state rift migration is capable of explaining the rifted margin formation of the Central South Atlantic segment and the Iberia/Newfoundland conjugates. Moreover, this process may be relevant for other hyper-extended and highly asymmetric margin pairs such as Antarctica–India [36] , the North-East Atlantic [37] , [38] , the Southern South Atlantic segment [39] and the East Australia/Lord Howe Rise conjugates [40] . Modelling techniques Using numerical thermo-mechanical modelling techniques [41] , we investigate the mechanism causing asymmetry and crustal hyper-extension during lithospheric thinning. Our models incorporate rheologies, initial temperature fields and extension velocities adequate for the Central South Atlantic segment and West Iberia–Newfoundland. Importantly, our simulations are strictly based on experimental rheological data for major rock types. By computing the degree of partial melting in the mantle, we ensure that our models are applicable to magma-poor margins: All shown models predict melt equivalent to <1.5 km of magmatic underplate before crustal break-up. Numerical techniques The forward models of rift evolution have been conducted using a 2D version of the finite-element code SLIM3D [41] (Semi-Lagrangian Implicit Model for 3 Dimensions), which has been successfully applied to model geodynamic processes at divergent [25] , [42] , [43] , [44] , convergent [45] , [46] and transform [47] plate boundaries. The programme relies on the Arbitrary Lagrangian-Eulerian Method to solve the thermo-mechanically coupled conservation equations of momentum, energy and mass. Re-meshing is conducted in order to track the motion of the free surface and to avoid large grid distortion. During re-meshing, we use the particle-in-cell method in order to resolve advection of the material phases and history variables, such as accumulated plastic strain. SLIM3D involves an elasto-visco-plastic rheology formulation by adopting an additive decomposition of the deviatoric strain rate into elastic, viscous and plastic components. This approach allows to reproduce a wide range of lithospheric deformation processes such as faulting, flexure and lower crustal flow. The viscous strain rate component simultaneously accounts for two creep mechanisms: diffusion and dislocation creep. Brittle deformation is incorporated using the Mohr–Coulomb failure model. Moreover, SLIM3D includes full compressibility, linear elasticity, shear heating, viscous and frictional strain softening, and power-law related strain rate softening. A setup sketch and a table with all model parameters are provided in Supplementary Fig. 1 and Supplementary Table 1 , respectively. All shown models are computed within a 2D domain that is 500 km wide and 150 km deep. Lateral and vertical element size is 1 km, resulting in 75,000 elements and ~\n150,000 nodes. We use time steps of 10 ky and let the model evolve over 40 My unless otherwise indicated. The present version of SLIM3D solves the discretized conservation equations using the direct parallel shared memory solver PARDISO [48] . Thermal model setup The initial thermal state of the model is the equilibrated temperature distribution that results from layer-specific heat conductivity, radiogenic heat production and the following boundary conditions: the surface temperature is held constant at 0 °C. Below 120 km depth (unless otherwise indicated), the asthenosphere temperature is set to 1,300 °C. Lateral boundaries are thermally isolated. A small thermal heterogeneity is introduced in the model centre in order to avoid rift localization at the model boundaries. This heterogeneity is generated by elevating the initial 1,300 °C isotherm in form of a triangular shape with a 5-km height and 20-km width (see Supplementary Fig. 1 ). During subsequent model evolution, we fix the bottom boundary temperature to 1,300 °C. The chosen depth of 120 km for the initial thermal LAB boundary (that is, the 1,300 °C isotherm) is based on compiled present day data for African Mobile belts [34] . Note that present day lithosphere thickness in Iberia and Newfoundland is somewhat smaller than at the South Atlantic conjugates [34] , which is reflected in our models by using a 105-km initial lithospheric thickness. However, the low magmatic activity of the rifts indicates relatively cold pre-rift geotherms. Our models feature an initial surface heat flow of 63 and 67 mW m − 2 for the South Atlantic and Iberia–Newfoundland setup, respectively, with corresponding initial Moho temperatures of 550 °C and 600 °C. Available quantitative inferences from an exposed Alpine magma-poor margin indicate pre-rift Moho temperatures of 550–650 °C [49] . Melt generation We compute magma generation in a post-processing step using a batch-melting model for peridotite [50] . The solidus temperature for a given pressure is T sol =−5.1 p 2 +132.9 p +1,085.7, whereas the liquidus temperature is T liq = −3.2 p 2 +80.0 p +1,475. Hereby, temperatures are measured in °C and pressure p in GPa. After computing T sol and T liq at each element, we quantify the melt fraction of peridotite X at the temperature T as X =(( T−T sol )/( T liq −T sol ) ) 3/2 . We account for endothermic consumption of lattice energy by computing the associated temperature change Δ T lattice =X Δ S/C p ( T+ 273), with the entropy change during melting [50] Δ S =300 J kg −1 K −1 and the heat capacity C p =1,200 J kg −1 K −1 (see Supplementary Table 1 ). We evaluate the melt fraction that is self-consistent with lattice energy consumption by iterative computation of X and T=T 0 − Δ T lattice , where T 0 is the initial temperature that does not account for energy consumption during melting. Vertical integration over the melt-generating area allows us to approximate how much magma is produced by decompression melting. Even if we assume that all melts reach the surface, which is certainly an end member scenario, our model in Fig. 1 indicates up to 0.8 km of melt thickness before crustal break-up, thus illustrating the applicability of our model to magma-poor margins. The post-break-up melt thickness of 1.2 km agrees with observed thickness of the oceanic crust at ultra-slow (<12 mm per year full spreading rate) spreading ridges [51] , especially if one considers that in reality not all melt reaches the surface. We have tested the effect of a higher asthenosphere temperature (1,350 °C) on model evolution. Depending on extension velocity, melt thickness increases up to several kilometres, comparable to the high-velocity layer described at the Angolan margin [3] . However, the overall model outcome and particularly our conclusions concerning the influence of extension velocity, thermal LAB thickness and initial fault configuration remain robust. Rheological model setup Our model involves four distinct petrological layers (upper and lower crust, strong and weak mantle). The upper crustal layer is 22 km thick and deforms in accordance with a wet quartzite flow law [52] . The mafic crust between 22 and 33 km depth deforms via a wet anorthite flow law [53] . Evidence for the rheology of the lower crust derives from seismic studies that feature P-wave velocities within the lower crust >6.6 km s −1 at the Iberia–Newfoundland conjugates [16] , [54] , [55] , [56] and >6.7 km s −1 in Angola [3] , which provides strong evidence for a mafic composition [57] . Independent evidence comes from Alpine geology, where the exposed lower crust of the Adriatic plate is rich in granulites and mafics [58] . The initial Moho depth of 33 km is supported by seismically inferred crustal thickness in Iberia [59] , Newfoundland [54] and Brazil [60] . Thirty-three kilometres crustal thickness corresponds to pressures of 0.9 GPa at the base of the crust. This value agrees with mineral chemistry studies [49] of obducted passive margins in the Alps that indicate pre-rift Moho pressures of ~\n0.9±0.1 GPa. We use dry olivine rheology [61] to model deformation of the strong, depleted, subcontinental mantle, whereas we use a wet olivine (that is, 500 p.p.m. H/Si) flow law [61] for the weak, asthenospheric mantle. We assume a grain size of 6 mm that is included in the pre-exponential factors. The boundary between weak and strong mantle initially resides 30 km above the thermal LAB boundary, that is, the 1,300 °C isotherm because weak mantle material cools and attaches (freezes) onto the mechanically strong mantle layer until Rayleigh–Taylor instabilities evolve. Our initial condition is consistent with long-term thermo-mechanical equilibration [62] . Weakening mechanisms Besides shear heating and dislocation creep-related strain rate softening, the model accounts for two mechanical weakening mechanisms that have been observed in laboratory and nature [63] , namely friction softening and viscous softening that are discussed below. Frictional softening is responsible for localization of faults [64] , and is incorporated in our model by a dependency of the friction coefficient on accumulated plastic strain. The unstrained initial friction coefficient of 0.5 is thereby linearly reduced to 0.05 for accumulated plastic strain of 1. If strain exceeds 1, the friction coefficient remains constant at 0.05. In laterally homogeneous models with symmetric boundary conditions, the whole model evolution should remain symmetric. This permanent symmetry is a model artefact as lateral homogeneity does not exist in natural settings because of inherited structures such as crustal faults. In our model, we therefore introduce lateral heterogeneity by applying a small arbitrary variation to the initial friction coefficient at each numerical element. This procedure results in a random distribution of initial friction coefficients that varies between 0.4 and 0.5. In our model, the orientation of faults and thus the asymmetry of the developing rift is not prescribed and generates spontaneously. Viscous strain softening leads to localization in ductile material. This weakening mechanism relates to the fact that large strains cause grain-size reduction in ductile shear zones [65] , [66] possibly via dislocation creep and dynamic recrystallization. Low grain size, however, facilitates deformation by grain-size sensitive diffusion creep leading to a switch in deformation mechanism that involves severe viscosity reduction [67] , [68] . We use a simple parameterization for viscous strain softening by linearly increasing the pre-exponential factor in the strain rate to stress relation of the dislocation flow law. Between a viscous strain of 0 and 1, the pre-exponential factor increases by a factor f . In our models, we use f =30 that implies a change in viscosity by a factor of 30 −1/ n , where the stress exponent n ranges between 3 (wet anorthite [53] , lower crust) and 4 (wet quartzite [52] , upper crust). Hence, this procedure generates a modest viscosity decrease between 0.3 and 0.4 compared with unstrained material. Mechanical boundary conditions Rifting is induced by prescribing a velocity of 4 mm per year at lateral boundaries, resulting in a full extension velocity of 8 mm per year, unless otherwise indicated. The free surface boundary condition at the top of the model allows self-consistent evolution of topography. At the bottom boundary, isostatic equilibrium is realized by means of the Winkler foundation [41] . Alternative numerical model setups In order to test the robustness of our results, we conducted a series of experiments with alternative model setups where we varied the size of the computational domain and the numerical resolution, we introduced a free slip condition at the lower model boundary and applied the full extensional velocity at only one side of the model. Despite small differences between all models, the overall results of this study remain unchanged. We also checked whether serpentinization would influence our results. We introduced a phase change from olivine to serpentine using a pressure- and temperature-dependent serpentine stability field [17] , [69] . We found that serpentinization does not occur near the exhumation channel owing to its elevated temperatures. According to our simulations, it takes place only before break-up and therefore does not have a qualitative influence on our conclusions. South Atlantic plate kinematics The South Atlantic Rift velocities and margins width ( Fig. 3 ) have been computed using a new plate kinematic model for the separation of South America and Africa [24] . The model quantitatively integrates crustal deformation from Cretaceous African and South American intraplate deforming zones, as well as from the South Atlantic conjugate passive margins. How to cite this article: Brune, S. et al. Rift migration explains continental margin asymmetry and crustal hyper-extension. Nat. Commun. 5:4014 doi: 10.1038/ncomms5014 (2014).